Identification and design principles of low hole effective massp-type transparent conducting oxides The development of high-performance transparent conducting oxides is critical to many technologies from transparent electronics to solar cells. Whereas n -type transparent conducting oxides are present in many devices, their p -type counterparts are not largely commercialized, as they exhibit much lower carrier mobilities due to the large hole effective masses of most oxides. Here we conduct a high-throughput computational search on thousands of binary and ternary oxides and identify several highly promising compounds displaying exceptionally low hole effective masses (up to an order of magnitude lower than state-of-the-art p -type transparent conducting oxides), as well as wide band gaps. In addition to the discovery of specific compounds, the chemical rationalization of our findings opens new directions, beyond current Cu-based chemistries, for the design and development of future p -type transparent conducting oxides. Transparent conducting oxides (TCOs) are compounds exhibiting high electrical conductivity and transparency to visible light. Those materials are needed in many applications from solar cells, where a TCO thin film provides electrical contact without impeding the flux of visible light reaching the device, to transparent transistors that could, for instance, be integrated in windows [1] , [2] , [3] , [4] , [5] . The main strategy to achieve the two antagonistic properties of high conductivity and transparency is to use wide band gap oxides (favouring transparency) doped with a significant amount of mobile charge carriers, either holes ( p -type) or electrons ( n -type) [6] . n -TCOs (for example, indium tin oxide) are already present in many modern devices but p -TCOs have not been largely commercialized, as their carrier mobilities stand an order of magnitude behind their n -counterparts. This situation impedes many critical technological developments from more efficient organic and thin film solar cell designs, benefiting from a better band matching by using p- instead of n -TCOs [7] , [8] , to the entire new field of transparent electronics that requires both p- and n -type TCO materials [2] , [9] , [10] , [11] , [12] , [13] . There is a fundamental reason to the difficulty of developing high-mobility p -type TCOs: the localized oxygen p nature of the valence band in most oxides makes those bands very flat and leads to large hole effective masses [12] , [13] . The field of p -type TCOs received most of its impulse a decade ago when Kawazoe et al. [14] demonstrated that CuAlO 2 delafossite could show encouraging p -type conductivity and optical transparency in visible light [14] . The unusual hole mobility of CuAlO 2 was explained by a large hybridization of the oxygen orbitals with 3 d 10 electrons in the Cu 1+ closed shell, lowering the oxygen character and leading to dispersive (low effective mass) valence band. This finding led to the outline of a design rule for p -type TCOs requiring the presence of Cu 1+ and motivated the study of a very large range of Cu-based materials [12] , [13] such as other delafossites (for example, CuCrO 2 (ref. [15] 15), SrCu 2 O 2 (refs [16] , [17] 16,17) or Cu-based oxychalcogenides [18] ). To this day, the question remains open whether alternative chemistries and design rules could lead to materials with lower hole effective mass. Answering this question is critical for the p -type TCO field, as it would enable the identification of the high hole mobility oxides that the TCO community has been looking for. In this work, we use a high-throughput ab initio computational approach to browse the electronic structure for thousands of binary and ternary oxides [19] , [20] , [21] . We identify the compounds and chemistries leading to low hole effective mass and wide band gap materials and propose several novel p -type TCO candidates. In addition to the identification of specific compounds, we discuss the underlying chemical reasons for those exceptionally low hole effective masses and propose novel design rules for the development of p -type TCOs. Distribution of electron and hole effective masses Our database contains density functional theory (DFT) band structures for 3,052 oxides. All the oxides are existing minerals, or already synthesized materials, whose experimentally measured crystalline structure has been taken from the Inorganic Crystal Structure Database (ICSD) ( http://www.fiz-karlsruhe.de/icsd.html ). We have taken their first principles relaxed crystalline structure as available in the Materials Project Database ( http://www.materialsproject.org ) [22] and computed their electronic structure (band gaps and effective masses) using state-of-the-art methodologies, as described in the Methods section. 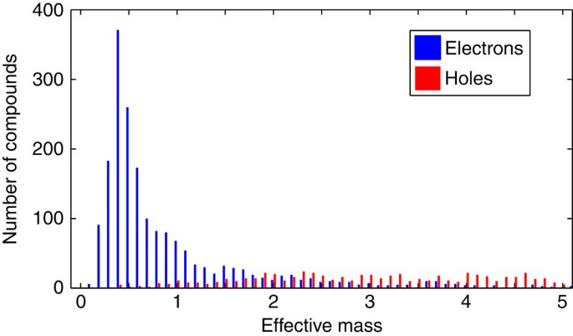Figure 1: Effective mass distribution for electrons and holes in oxides. The histogram shows the maximum line effective mass for holes (valence band) in red and electrons (conduction band) in blue in our set of binary and ternary oxides. The effective mass bin size is 0.2 and the figure focuses on the region of low effective mass (lower than 5). Figure 1 shows the histogram of hole (in red) and electron (in blue) effective masses. The difference in distribution between hole and electron effective masses is striking, emphasizing that finding high-mobility p -type oxides is indeed significantly more challenging than finding n -types. The chemical reasons for such a difference comes from the very different character of the valence and conduction bands in oxides. The valence bands tend to be of localized oxygen p character (leading to large effective masses) whereas the conduction bands are cationic and more often dispersive (leading to low effective masses) [23] , [24] . Figure 1: Effective mass distribution for electrons and holes in oxides. The histogram shows the maximum line effective mass for holes (valence band) in red and electrons (conduction band) in blue in our set of binary and ternary oxides. The effective mass bin size is 0.2 and the figure focuses on the region of low effective mass (lower than 5). Full size image Low hole effective mass and large band gap oxides Although low hole effective mass oxides are rare, our large database offers the opportunity to identify the outliers. Searching for compounds with exceptionally low effective mass (<1.5), we identify 20 oxides that have never been considered as TCOs. Details on the screening procedure are available in the Methods section. To further assess the practical interest of the TCO candidates, we also evaluate their band gaps, as this would influence their light absorption. As DFT does not model band gaps as accurately as band shapes and widths, we compute band gaps with a higher order method: many body perturbation theory in the GW approach [25] , [26] . The band structure of each candidate is presented in Supplementary Figs S1–S20 . 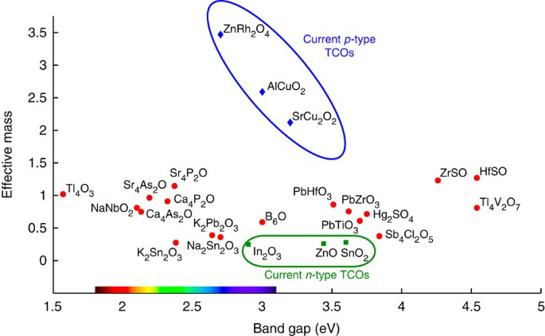Figure 2: Effective mass versus band gap for thep-type TCO candidates. We superposed on the band gap axis a colour spectrum corresponding to the wavelength associated with a photon energy. The TCO candidates are marked with red dots. A few knownp-type (blue diamonds) andn-type (green square) TCOs can be compared to the new candidates. The best TCOs should lie in the lower right corner. For clarity, we kept only one representative when polymorphs existed for a given stoechiometry (for example, PbTiO3and K2Sn2O3) and did not plot Rb2Sn2O3, which is superposed on K2Sn2O3. Figure 2 plots the effective mass versus the band gap for the 20 identified compounds (red dots). For comparison, we also plot a few known p -type TCOs (blue diamonds, Cu-based TCOs and ZnRh 2 O 4 ) and some current n -type materials (green squares, SnO 2 , In 2 O 3 and ZnO). The data are also available in Supplementary Tables S1–S4 . The compounds we have identified beat the state-of-the-art p -type TCOs by up to an order of magnitude in effective mass. Some compounds are even reaching hole effective mass values close to the best electron effective mass exhibited by current n -type oxides. This shows that the large difference in mobility between current n -type and p -type materials is not inevitable and could be overcome by the investigation of alternative chemistries. Figure 2: Effective mass versus band gap for the p -type TCO candidates. We superposed on the band gap axis a colour spectrum corresponding to the wavelength associated with a photon energy. The TCO candidates are marked with red dots. A few known p -type (blue diamonds) and n -type (green square) TCOs can be compared to the new candidates. The best TCOs should lie in the lower right corner. For clarity, we kept only one representative when polymorphs existed for a given stoechiometry (for example, PbTiO 3 and K 2 Sn 2 O 3 ) and did not plot Rb 2 Sn 2 O 3 , which is superposed on K 2 Sn 2 O 3 . Full size image The best TCOs should lie in the lower right corner, as they would show small effective masses and large band gaps. However, the materials containing toxic elements such as Pb, Tl and Hg are less likely to be of interest technologically. The series of A 4 B 2 O oxypnictides compounds ( A =Ca, Sr and B =P, As) and NaNbO 2 are not of high priority, as compounds with both higher band gaps and lower effective masses are present in our data set. K 2 Sn 2 O 3 (rhombohedral or bcc) and Rb 2 Sn 2 O 3 show the lowest effective mass around 0.27–0.28 but a band gap on the small side (2.4 eV). Interestingly, the band gap of K 2 Sn 2 O 3 can be increased by substituting Na that would lead to lower absorption in the visible (see Supplementary Note 1 and Supplementary Fig. S21 ). K 2 Pb 2 O 3 also possesses a higher band gap than K 2 Sn 2 O 3, with similar effective masses but with the drawback of Pb toxicity. On the other hand, the ZrOS and HfOS compounds have larger effective masses but with a significantly larger band gap and opportunities for full visible range transmission. Finally, both Sb 4 Cl 2 O 5 and B 6 O have large band gaps (respectively, 3.6 and 3 eV) and low effective masses (respectively, 0.37 and 0.59). We performed our analysis using the electronic band gap, but forbidden optical transitions can make the optical band gap significantly larger, as is the case in In 2 O 3 (ref. 27 ). Thus, we have also computed all the optical absorption spectra (see Supplementary Fig. S22 ). None of the smaller electronic gap materials (<3 eV) show an optical gap significantly higher than their electronic gap. Hence, the conclusions drawn from the electronic band gap still hold. p -type dopability of the most promising candidates A low hole effective mass and a large band gap are necessary for any high-performance p -type TCO and it is remarkable that those two simple constraints already exclude the vast majority of known oxides (>99%). However, the possibility to generate holes in the valence band (that is, the p -type dopability) is not guaranteed a priori for our candidates. It is indeed well reported that most oxides have fundamental thermodynamic constraints, making their p -type doping difficult [28] , [29] , [30] . More specifically, the formation of compensating intrinsic defects (hole killers) such as the oxygen vacancy when lowering the Fermi energy towards the valence band has been identified as the main impediment to p doping in oxides. Whereas none of our candidates have ever been tested (or even suggested) as TCOs, doping studies indicating p -type dopability have already been reported experimentally or computationally for several of them. B 6 O has been experimentally measured to show p -type conductivity [31] . It has been demonstrated experimentally that PbZr 0.5 Ti 0.5 O 3 can be grown as p -type [32] , but some recent computations on PbTiO 3 seem to indicate an oxygen vacancy low in energy even in oxidizing conditions [33] . Finally, a recent computational study on ZrOS defects demonstrated that the oxygen vacancy is not a hole killer in oxidizing conditions (to the contrary of ZrO 2 ) [34] . For the remaining chemistries of greatest interest, we perform defect computations (see Methods), focusing on all the vacancy intrinsic defects as in Trimarchi et al. 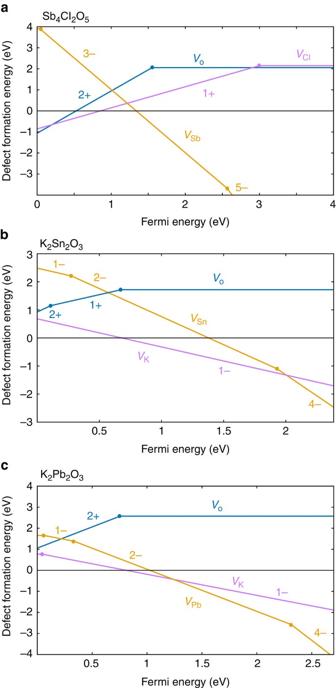Figure 3: Vacancy formation energy versus Fermi energy. The panels indicate results for Sb4Cl2O5(a) K2Sn2O3(b) and K2Pb2O3(c). The oxygen vacancy formation energy is indicated by a blue line. The cation vacancies are indicated by orange and purple lines. All defects are calculated in oxidizing conditions. The zero of Fermi energy is the valence band maximum. [35] Figure 3 shows the defect-formation energy as a function of the Fermi energy for Sb 4 Cl 2 O 5 , K 2 Sn 2 O 3 and K 2 Pb 2 O 3 in oxidizing conditions (most favourable for p -type behaviour). Figure 3a shows that Sb 4 Cl 2 O 5 is not likely to be p -type doped. Indeed, when the Fermi energy is close enough to the valence band to generate holes, compensating defects (that is, oxygen and chlorine vacancies) will form spontaneously and act as hole killers. On the other hand, for K 2 Sn 2 O 3 ( Fig. 3b ), the oxygen vacancy will not compensate hole formation. Moreover, the presence of a low-energy potassium vacancy can lead to intrinsic p -type behaviour for this material. This behaviour is similar to the defect energetics in known p -type oxides such as Cu 2 O (ref. 36 ), or CuAlO 2 (ref. 37 ). K 2 Pb 2 O 3 shows a similar behaviour (see Fig. 3c ) as well as the other bcc phase of K 2 Sn 2 O 3 (see Supplementary Fig. S23 ). These results demonstrate that all our most promising candidates (apart from Sb 4 Cl 2 O 5 ) do not only combine low hole effective masses and wide band gap but have also defect energetics favouring p -type behaviour. The determination of the exact amount of hole carriers that those materials could be doped with (intrinsically or extrinsically) will require future experimental and theoretical work. Both high hole and low hole concentrations are of interest, depending on the application. In devices such as solar cells, where high hole conductivity is sought for, we typically look for high hole concentration TCOs. However, other devices such as transparent transistors typically require TCOs with lower hole concentrations [38] . Figure 3: Vacancy formation energy versus Fermi energy. The panels indicate results for Sb 4 Cl 2 O 5 ( a ) K 2 Sn 2 O 3 ( b ) and K 2 Pb 2 O 3 ( c ). The oxygen vacancy formation energy is indicated by a blue line. The cation vacancies are indicated by orange and purple lines. All defects are calculated in oxidizing conditions. The zero of Fermi energy is the valence band maximum. Full size image Our approach has led to the identification of several new p -type TCO candidates but the results can also be analysed to understand the inherent chemical principles leading to low hole effective masses. 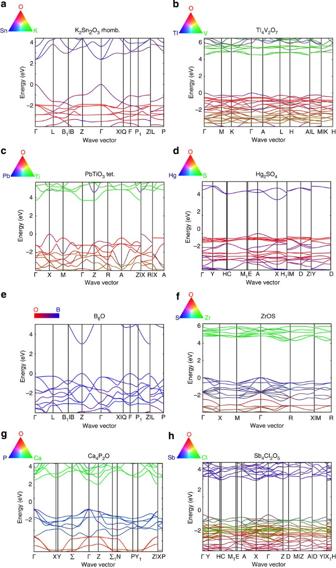Figure 4: Projected band structures for low hole effective mass oxides. The panels refer to K2Sn2O3rhombohedral (a), Tl4V2O7(b), PbTiO3tetragonal (c), Hg2SO4(d), B6O (e), ZrOS (f), Ca4P2O (g), Sb4Cl2O5(h). The band structures are computed by GGA with a rigid shift of the conduction band (scissor operator) to fit the band gap to theGWvalue. The colour indicates the character of the bands by projections of the wave function on the different sites. Each element in the ternary compound has one of the red, green or blue colour associated with it and the resulting colour is obtained by mixing them in proportion equivalent to the projections. The red colour is always associated with oxygen. Equivalent Figures without colour scheme but with markers are available inSupplementary Figs S24–S31. Figure 4 shows the band structure of one representative of each of the chemistries identified (K 2 Sn 2 O 3 , Ca 4 P 2 O, Tl 4 V 2 O 7 , PbTiO 3 , ZrOS, B 6 O and Sb 4 Cl 2 O 5 ). The colour scheme indicates the nature of the band obtained by projecting the wave functions on the different elements. For the ternary compounds, one of the red, green or blue colours is associated with the different elements and the resulting colour is obtained by mixing those primary colours proportionally to the projections. The red colour is always associated with oxygen. For the only binary B 6 O, red is used for oxygen and blue for boron. All compounds have dispersive valence bands, with a high curvature near the valence band maximum, indicative of a low hole effective mass. For all of them, the oxygen character of the valence band is mild, in agreement with the localized nature of oxygen 2 p orbitals. Whereas our candidates cover different chemistries, the low-effective-mass valence bands can be explained by two main mechanisms that are both related to a chemical way of producing valence bands with low oxygen character. Figure 4: Projected band structures for low hole effective mass oxides. The panels refer to K 2 Sn 2 O 3 rhombohedral ( a ), Tl 4 V 2 O 7 ( b ), PbTiO 3 tetragonal ( c ), Hg 2 SO 4 ( d ), B 6 O ( e ), ZrOS ( f ), Ca 4 P 2 O ( g ), Sb 4 Cl 2 O 5 ( h ). The band structures are computed by GGA with a rigid shift of the conduction band (scissor operator) to fit the band gap to the GW value. The colour indicates the character of the bands by projections of the wave function on the different sites. Each element in the ternary compound has one of the red, green or blue colour associated with it and the resulting colour is obtained by mixing them in proportion equivalent to the projections. The red colour is always associated with oxygen. Equivalent Figures without colour scheme but with markers are available in Supplementary Figs S24–S31 . Full size image The first mechanism leading to compounds with low effective masses and wide band gaps concerns K 2 Sn 2 O 3 , Rb 2 Sn 2 O 3 , PbTiO 3 , PbZrO 3 , PbHfO 3 , K 2 Pb 2 O 3 , Tl 4 O 3 and Tl 4 V 2 O 7 ( Fig. 4a–d ). For these compounds, the low hole effective mass originates from the hybridization of the s states of a (n−1) d 10 n s 2 cation (for example, Sn 2+ , Pb 2+ or Tl 1+ ) with oxygen 2 p orbitals. This is similar to what happens for Cu-based compounds in which the closed 3 d shell is hybridized with oxygen. However, s orbitals are significantly more delocalized than d orbitals, leading to higher dispersion of the valence band and lower effective masses (up to an order of magnitude as shown in Fig. 2 ). The impact of (n−1) d 10 n s 2 ions on the valence-band shape in oxides has been already discussed in other fields such as photocatalysis [39] , [40] but has not been much used for the design of p -type TCOs. So far, the only studied (n−1) d 10 n s 2 ion p -type oxide has been SnO [41] , [42] . However, SnO suffers from a very small indirect gap (0.7 eV) [42] and its valence band shows anisotropic effective mass because of its layered structure. Our work shows that going to ternary oxides of Sn 2+ can lead to wider band gaps (similarly than going from Cu 2 O to CuAlO 2 widens the gap of Cu-based compounds) but also to more isotropic effective masses by modifying the crystal structure. The Hg 2 SO 4 compound also shows an orbital overlap of s electrons with oxygen p even if Hg 1+ has a slightly different electronic configuration 5 d 10 6 s 1 . From our set of (n−1) d 10 n s 2 -containing compounds, we found that the oxygen hybridization is most pronounced for Sn 2+ followed by Pb 2+ and finally Tl 1+ , which has the least dispersive valence bands and the strongest oxygen character. Whereas Bi 3+ is also (n−1) d 10 n s 2 and some Bi-based compounds were close to meet our criteria (for example, BiVO 4 , Bi 2 Ti 4 O 11 and BiBrO, see Supplementary Table S1 ), none of them passed the 1.5 cutoff on average effective mass. It is possible that our data set did not contain the adequate crystal structure to lead to large bismuth s -oxygen p overlap in every directions, although such a structure might be achievable. A Sb 3+ -based compound (Sb 3+ is 4 d 10 5 s 2 ) is also present in our candidates (that is, Sb 4 Cl 2 O 5 ). However, here not only does the s orbital of Sb hybridize with oxygen, but the valence band character is also influenced by the presence of anionic chlorine. The presence of an additional anion is actually the second mechanism at play in our low-effective-mass candidates (that is, ZrOS, HfOS and the oxypnictides) as illustrated by the bands characters presented in Fig. 4e–h . Here the valence band keeps a p character but more delocalized orbitals such as 3 p (for S 2− , P 3− ) or 4 p (As 3− ) replace the oxygen 2 p valence band. Although pure 3 p- or 4 p -based compounds have often too small band gaps, the mixing of oxygen and another p -orbital anion can lead to compounds with low effective masses and large band gaps. For instance, the band gaps of ZrS 2 is 1.7 eV (ref. 43 ), whereas ZrO 2 shows a larger band gap (from 5.2 to 5.7 eV (ref. 44 )) but flat oxygen valence bands. ZrOS achieves an interesting trade-off offering a larger band gap than for the pure sulphide with a lower hole effective mass because of the sulphur character of the valence band. Our study did not lead to any oxypnictides offering such a good trade-off, but it is a still unexplored chemistry where future TCO work might be fruitful. Boron suboxide also fits in the anion-mixing category, as B 6 O can be seen as a mixture of cationic boron, anionic boron and anionic oxygen. Knowing the rarity of p -type oxides, it is fortunate that the majority of our low hole effective mass candidates show either experimental or computational evidence for p -type dopability. This not a coincidence, as both mechanisms at play (hybridization of oxygen with (n−1) d 10 n s 2 or mixing of oxygen with another anion) lead to higher valence band energies than typical oxides, which induces easier p -type doping [28] , [29] , [30] . In summary, we have studied a large database of computed band structures for thousands of oxides, searching for the chemistries prone to low-effective-mass oxides. Our large-scale study confirms that holes tend to have higher effective masses than electrons in oxides, but it identifies several compounds with exceptionally low hole effective masses and wide band gaps. Further analysis on p -type dopability suggests a few novel earth-abundant, p -type TCO candidates: B 6 O, A 2 Sn 2 O 3 (A=K, Na), ZrOS, as well as the less environmentally friendly PbTiO 3 and K 2 Pb 2 O 3 . By analysing those results, two novel design principles, leading to compounds with lower effective masses than state-of-the-art p -type TCOs, emerge: hybridization of a (n−1) d 10 n s 2 (especially Sn 2+ and Pb 2+ , but also Bi 3+ or Sb 3+ ) with oxygen and/or the presence of an anion with p -orbitals more delocalized than oxygen (for example, S 2− , P 3− , Cl − or Br − ). Those principles are extremely valuable to guide future searches for high-mobility p -type TCO and, after a decade of exploration of Cu-based chemistries, they offer new chemical spaces full of promises. High-throughput computations and screening All the high-throughput DFT computations were performed using the Vienna software package (VASP) [45] , with PAW pseudopotentials [46] and the generalized gradient approximation (GGA) as implemented by Perdew, Burke and Ernzerhoff (PBE) [47] . We considered all compounds containing less than 100 atoms in the unit cell present in the Materials Project database (http://www.materialsproject.org) [22] originally from the ICSD ( http://www.fiz-karlsruhe.de/icsd.html ) and containing oxygen and no elements such as rare-earths (from Z=58, Ce to Z=71, Lu), inert gases and any element with an atomic number larger than 84 (Po). All ionic relaxations in the Materials Project Database were performed using AFLOW [48] with the high-throughput computation parameters described in Jain et al. [22] For the high-throughput band structure computations, we used the Materials Project structures (already relaxed with GGA) and performed a static run to obtain the charge density, followed by a non-self-consistent band structure run along the band structure symmetry lines provided by Curtarolo et al. [19] , [48] Our screening procedure consisted of evaluating first the effective mass along the band-structure symmetry lines. If none of those were higher than 1.5, we also performed a full average effective mass tensor computation on a regular Γ-centred 8,000 k -points grid interpolated using the Boltztrap code [49] . This average effective mass tensor takes into account effects of non-parabolicity, multiple bands, multiple minima and anisotropy. More details on the average effective mass and the screening procedure are given in Supplementary Methods (with a flow chart in Supplementary Fig. S32 ). All data analyses (for example, effective mass computations or band structure plotting) were carried out using the pymatgen python package [50] . GW computations In the one-shot GW (or G 0 W 0 ) approach, corrections are obtained perturbatively from a starting DFT electronic structure. GW and preparatory DFT calculations on the 20 target compounds were performed with the ABINIT code [51] at optimized geometries, obtained from the Materials Project database. The exchange correlation energy for the preparatory DFT computation was described using the local density approximation functional [52] . The Brillouin Zone was sampled with Monkhorst–Pack grids and the k -point sampling density was similar for all considered systems (>450/ n k -points, where n is the number of atoms in the unit cell). For each oxide, the planewave cutoff was determined separately and set using a total energy difference convergence criterion, leading to electronic energies converged within 10 −3 eV on average. We used norm-conserving pseudopotentials to model the electron-ion interaction. If any, we included semi-core d states as valence in the pseudopotential. Supplementary Table S5 gives details on the pseudopotential used. The GW calculations were carried out using the well-established Godby–Needs plasmon pole approximation [53] . The accuracy of some other plasmon pole approximations has been recently questioned. However, the Godby–Needs plasmon pole approximation has been shown to give the same results as the full contour deformation numerical integration for several oxides [54] [55] . We used a cutoff of 20 Rydberg for the expansion of the dielectric matrix and performed convergence studies with respect to number of bands for all our candidates. The band gaps are converged within 0.1 eV (up to 1,300 bands are needed). While considering the GW band gaps, the reader should keep in mind that the G 0 W 0 approach that we use, although significantly more predictive than DFT, nevertheless still slightly underestimates band gaps (by around 0.2 eV in average) [26] . Absorption spectra computations The absorption coefficient computations followed the methodology from Yu et al. [56] and used the random phase approximation approach as implemented in VASP on the GGA band structure [57] . No phonon-assisted transition or excitonic effects were taken into account but a scissor shift resulting from the GW calculations was applied to the GGA results. A Monkhorst-Pack grid of at least 10 × 10 × 10 k -points and a number of bands three times larger than for the ionic relaxation were used for all computations. Defect computations All defect computations were performed with a 2 × 2 × 2 k -point Monkhorst-Pack grid, with GGA-PBE on supercells (2 × 2 × 2 for K 2 Sn 2 O 3 and K 2 Pb 2 O 3 ; 3 × 2 × 1 for Sb 4 Cl 2 O 5 ). We used the electrostatic correction scheme provided by Freysoldt [58] . The defect energies were also corrected to take into account band-filling errors [59] . Finally, the band gap was corrected by shifting the valence and conduction bands by their bulk GW corrections while moving along the shallow defects with their band edge (that is, with the VBM for shallow acceptors) [59] . The chemical potential were obtained by computing the chemical potential region of stability for the compound with respect to all the compounds present in Materials Project database using the pymatgen package (see Supplementary Figs S33−S35 ) [50] . We selected the conditions of highest and lowest possible oxygen chemical potential for the given phase. Results for reducing conditions are available in Supplementary Figs S23 and S36−S38 . How to cite this article: Hautier, G. et al. Identification and design principles of low hole effective mass p -type transparent conducting oxides. Nat. Commun. 4:2292 doi: 10.1038/ncomms3292 (2013).